Genome-wide transcriptome profiling of homologous recombination DNA repair Homologous recombination (HR) repair deficiency predisposes to cancer development, but also sensitizes cancer cells to DNA damage-inducing therapeutics. Here we identify an HR defect (HRD) gene signature that can be used to functionally assess HR repair status without interrogating individual genetic alterations in cells. By using this HRD gene signature as a functional network analysis tool, we discover that simultaneous loss of two major tumour suppressors BRCA1 and PTEN extensively rewire the HR repair-deficient phenotype, which is found in cells with defects in either BRCA1 or PTEN alone. Moreover, the HRD gene signature serves as an effective drug discovery platform to identify agents targeting HR repair as potential chemo/radio sensitizers. More importantly, this HRD gene signature is able to predict clinical outcomes across multiple cancer lineages. Our findings, therefore, provide a molecular profile of HR repair to assess its status at a functional network level, which can provide both biological insights and have clinical implications in cancer. Genomic instability is a hallmark of cancer cells [1] . To maintain genomic stability and ensure high-fidelity transmission of genetic information, cells have evolved a complex mechanism to repair DNA double-strand breaks (DSBs), the most deleterious DNA lesions, in an error-free manner through homologous recombination (HR) [2] , [3] . HR-mediated DNA repair deficiency predisposes to cancer development [4] , but also sensitizes cancer cells to DNA damage-inducing therapy such as radiation therapy and DNA-damage-based chemotherapy [5] . HR repair involves a variety of proteins that detect, signal and repair DSBs [2] , [3] . It is coordinated by many cellular responses, such as cell cycle checkpoint, transcriptional activation, epigenetic regulation and various post-translational modifications [6] , [7] . The number of genes known to be involved in HR repair is constantly expanding [8] , [9] . Therefore, it would be virtually impossible to use conventional single-gene approaches to identify every possible genetic alteration that might lead to HR deficiency. In this study, we implemented a transcriptional profiling-based approach to systematically identify common molecular changes associated with defective HR repair and generated an HR defect (HRD) gene signature. We further validated that the HRD gene signature predicted HR status and sensitivity to Poly(ADP-ribose) polymerase (PARP) inhibitors in human cancer cells. More importantly, we were able to use the HRD gene signature to identify mechanisms underlying resistance to PARP inhibitors and confirm rational combination therapies predicted to synergize with PARP inhibitors. We also explored the clinical relevance of the HRD gene signature in multiple independent patient data sets and found that it correlated with overall survival across tumour lineages. In summary, we identify a gene signature, which can be used both to predict defective HR repair and clinical outcome in cancer patients. Identification of an HRD gene signature To obtain a comprehensive molecular understanding of HR repair process, rather than taking a single-gene approach to analyse HR repair in cells, we utilized a genome-wide gene expression profiling approach to systematically measure the cellular transcriptome reprogramming in HR-deficient cells. We used MCF-10A cells, an immortal human mammary epithelial cell line of nonmalignant origin, to establish isogenic cell lines with deficiency individually in three independent HR repair genes: BRCA1 , RAD51 and BRIT1 ( MCPH1 ). These genes were chosen due to their regulation of HR repair at different steps via distinct mechanisms. BRCA1 plays a critical role in DNA damage response signalling and the initial step of HR repair, DSB end resection [1] , [10] . RAD51 is the key recombinase enzyme for homologous sequence searching and recombination [11] . BRIT1 mediates HR repair, likely through regulating chromatin structure [12] , [13] . As expected, the cell lines with deficiency in BRCA1 , RAD51 or BRIT1 had significantly reduced HR repair efficiency ( Supplementary Fig. 1a,b ). Importantly, all the knockdown cell lines exhibited cell cycle distribution similar to that of the control cells ( Supplementary Fig. 1c ), which excluded effects caused by changes in cell cycle progression. We then used microarray analysis to search for genes differentially expressed between control and HR-deficient cell lines. 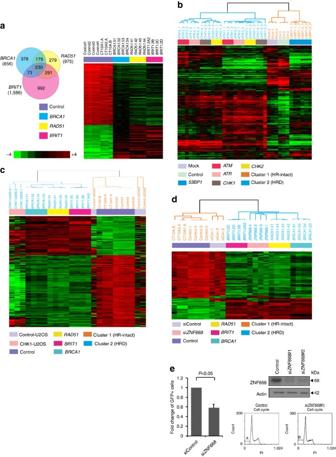Figure 1: Gene expression analysis identifies an HRD gene signature that functionally predicts the status of HR repair deficiency. (a) (Left) Venn diagram indicating numbers of genes whose expression differed between each HRD cell line and the other HRD cell lines and the control cells. The analysis was performed using BRB array tools. (Right) Heat map of the HRD gene signature, consisting of 230 genes whose expression differed between each HR-deficient cell line and the control cells. Microarray was conducted in seven independent samples of control cells and four independent samples of each individual knockdown cell line. Student’st-test was conducted between the average of control cells and that of knockdown cells (P<0.001). (b) MCF-10A cells were infected by lentiviral particles targetingATM,ATR,CHK1,CHK2or53BP1, and (c) U2OS cells were transfected by the ON-TARGET-plusCHK1siRNAs. Microarray analyses were conducted to verify accuracy and specificity of the HRD gene signature by supervised clustering analysis. (d) MCF-10A cells were transfected by the ON-TARGET-plusZNF668siRNAs. Microarray analysis was conducted to verify the presence of the HRD gene signature by supervised clustering analysis. (e) U2OS cells were transfected withZNF668siRNA or control siRNA and analysed for HR repair efficiency. Western blots demonstrating effective knockdown are shown to the upper right and cell cycle analysis with propidium iodide staining performed 72 h after transfection are shown to the lower right. We selected a set of 230 genes ( Supplementary Table 1 ) whose expression differed by a factor of two or more ( P <0.001) between each of the HR-deficient cell lines and parental cells ( Fig. 1a ) and designated the gene set as the HRD gene signature. As expected, a high proportion of genes in the HRD gene signature were involved in cell cycle regulation, DNA replication and DNA recombination and repair pathways ( Supplementary Fig. 2 ). In addition, a high proportion of genes in the HRD gene signature were in canonical pathways involved in mismatch repair, the function of BRCA1 and CHK proteins in DNA damage response, and cell cycle checkpoint control ( Supplementary Fig. 2 ). Importantly, expression of these genes is coordinately upregulated or downregulated in cell lines with HR deficiency induced by depletion of independent HR genes that have different mechanisms of action ( Fig. 1a ). For example, the expression levels of three DSB end resection enzymes, BLM , DNA2 and EXO1 , were all markedly reduced in HR-deficient cells, indicating DSB end resection efficiency would be expected to be correspondingly reduced by transcriptional regulation of resection enzymes. This observation showed that HR deficiency, independent of the specific mediator, leads to similar transcriptional changes. To exclude the possibility that the HRD gene signature is the result of cellular transcriptome reprogramming during stable selection, we further conducted transient transfection of BRCA1 small interfering RNA (siRNA) in MCF-10A cells and performed microarray analysis. Using supervised clustering analysis, we demonstrated that knocking down BRCA1 by siRNA in MCF-10A cells also led to the HRD gene signature ( Supplementary Fig. 3 ). All these findings strongly suggest that the molecular components involved in HR repair are interconnected and increases the likelihood that the HRD gene signature will capture defects in HR repair independent of the underlying mediator. Thus, it is possible that the HRD gene signature could allow for interrogation of the status of HR repair deficiency induced by multiple different mechanisms. Figure 1: Gene expression analysis identifies an HRD gene signature that functionally predicts the status of HR repair deficiency. ( a ) (Left) Venn diagram indicating numbers of genes whose expression differed between each HRD cell line and the other HRD cell lines and the control cells. The analysis was performed using BRB array tools. (Right) Heat map of the HRD gene signature, consisting of 230 genes whose expression differed between each HR-deficient cell line and the control cells. Microarray was conducted in seven independent samples of control cells and four independent samples of each individual knockdown cell line. Student’s t -test was conducted between the average of control cells and that of knockdown cells ( P <0.001). ( b ) MCF-10A cells were infected by lentiviral particles targeting ATM , ATR , CHK1 , CHK2 or 53BP1 , and ( c ) U2OS cells were transfected by the ON-TARGET-plus CHK1 siRNAs. Microarray analyses were conducted to verify accuracy and specificity of the HRD gene signature by supervised clustering analysis. ( d ) MCF-10A cells were transfected by the ON-TARGET-plus ZNF668 siRNAs. Microarray analysis was conducted to verify the presence of the HRD gene signature by supervised clustering analysis. ( e ) U2OS cells were transfected with ZNF668 siRNA or control siRNA and analysed for HR repair efficiency. Western blots demonstrating effective knockdown are shown to the upper right and cell cycle analysis with propidium iodide staining performed 72 h after transfection are shown to the lower right. Full size image The HRD gene signature predicts HR deficiency in cells To test this possibility, we first sought to determine whether the HRD gene signature was generalizable and able to predict HR deficiency induced by deficiency of independent HR-related genes. We generated gene expression profiles from isogenic MCF-10A cells with deficiency of various known key DNA damage response proteins, including ATM , ATR , CHK1 , CHK2 or 53BP1 (ref. 6 ) by both small hairpin RNA stable and siRNA transient knockdown. Using supervised clustering analysis, ATM -, ATR -, CHK1 - and CHK2 -deficient cells formed a cluster with the HRD gene signature ( Fig. 1b and Supplementary Fig. 4a,b ). In contrast, absence of the HRD gene signature was found in 53BP1 -deficient cells ( Fig. 1b and Supplementary Fig. 4a,c ). These observations are consistent with the well-established roles of the ATM-CHK2 and ATR-CHK1 pathways in regulating HR repair and the notion that 53BP1 functions as a negative regulator of DSB resection and HR repair. In order to demonstrate that such observations are not specific to MCF-10A cells, we established transient and stable CHK1 knockdown U2OS cells, which is a human osteosarcoma cell line and commonly used in the studies of DNA damage response and repair. CHK1 -deficient U2OS cells exhibited the same pattern of gene expression changes as those in the HRD gene signature derived from MCF-10A cells ( Fig. 1c and Supplementary Fig. 4b,d ). In addition, we generated a stable BRCA2 -deficient MCF-10A cell line, which also exhibited the HRD gene signature ( Supplementary Fig. 5a ). Consistent with this finding, two human breast cancer cell lines with BRCA2 mutations HCC1428 and HCC1369 showed the HRD signature pattern ( Supplementary Fig. 5b ). Collectively, these data demonstrated that the HRD gene signature differentiates HR-deficient cells from HR-intact cells and suggested that the HRD gene signature may represents a common molecular feature among different mechanisms or cell origins of generating HR deficiency. To further examine whether the HRD gene signature is functionally linked to HR repair-deficient status in cells, we tested whether it could determine genes with previously unknown function in HR repair are or are not involved in this process. We used zinc finger protein 668 ( ZNF668 ) as an example. ZNF668 was previously identified by genome-wide sequencing analysis as a frequently mutated gene in breast cancer [14] , [15] . However, molecular mechanisms underlying its tumour suppression function remains to be elusive. We conducted microarray analysis of ZNF668 -deficient cells and used supervised clustering to assess whether ZNF668 -deficient cells exhibited the HRD gene signature. Although individual HR repair factors such as BRCA1/2 , RAD51 , BRIT1 , ATM , ATR , CHK1 and CHK2 were not identified as top candidate genes based on expression changes in ZNF668 -knockdown cells, these cells clearly exhibited the HRD gene signature ( Fig. 1d ). HR repair assay showed that ZNF668 knockdown significantly impaired HR repair efficiency ( Fig. 1e ), without inducing any apparent difference in cell cycle distribution compared with control cells ( Fig. 1e ). We further knocked down ZNF688 in MDA-MB-436 breast cancer cells, which have a relative high expression level of ZNF668 compared with other breast cancer cell lines. We found that ZNF668 depletion significantly reduced RAD51 foci formation after IR treatment, without affecting cell cycle distribution ( Supplementary Fig. 6a,b ). In addition, we reconstituted ZNF668 expression in a breast cancer cell line EVSAT, which contains a ZNF688 nonsense mutation. We found that the restored expression of ZNF668 remarkably increased IR-induced RAD51 foci formation compared with control cells reconstituted with an empty vector with no apparent effect on cell cycle distribution ( Supplementary Fig. 6c,d ). These results indicated that the HRD gene signature can functionally link gene expression patterns with HR deficiency not only in our genetic engineered model systems but also various cancer cell lines, providing an opportunity to identify unexpected key players in HR repair. The HRD gene signature predicts PARP inhibitor sensitivity PARP inhibitors are recently identified targeted therapeutic drugs, which specifically kill HR repair-deficient cells via a synthetic lethality interaction [16] , [17] . As expected, BRCA1 -, RAD51 - and BRIT1 -deficient cells exhibited greatly increased cellular sensitivity to PARP inhibitor olaparib ( Supplementary Fig. 7a ). Thus, we reasoned that if the HRD gene signature is functionally linked to HR deficiency, it may serve as a powerful tool to predict the sensitivity of human cancer cells with diverse genetic backgrounds to PARP inhibitors. To test this possibility, we used two cell line panels: National Cancer Institute 60 (NCI60) [18] and a collection of 51 breast cancer cell lines [19] , which consist of cell lines from diverse human cancers that have been well characterized genetically and molecularly. Gene expression profiles of NCI60 ( Supplementary Fig. 7b ) and breast cancer 51 cell lines ( Supplementary Fig. 7c ) were clustered hierarchically into two groups on the basis of their similarity to the HRD gene signature. For prostate, renal, lung, ovarian and breast cancers, we selected HR-deficient and HR-intact cell lines as predicted by the HRD gene signature and determined HR repair efficiency using HR repair assay. Importantly, cell lines with the HRD gene signature showed reduced HR repair efficiency compared with their counterparts without the signature in each cancer type ( Fig. 2a ). Consistent with the results from the HR repair assay, cell lines with the HRD gene signature were more sensitive to PARP inhibitors olaparib ( Fig. 2b ) or rucaparib ( Fig. 2c ) treatment than cell lines with intact HR repair. It is very likely that PARP inhibitors will also be used in combination with standard DNA damaging agents in clinic. We, therefore, further tested whether cell lines with the HRD gene signature would be more sensitive to the treatment combining PARP inhibitors with temozolomide, a standard chemotherapy regimen. As shown in Supplementary Fig. 7d , consistent with the results from PARP inhibitor monotherapy, the HR-deficient cell line showed enhanced sensitivity compared with the HR-intact cell line. 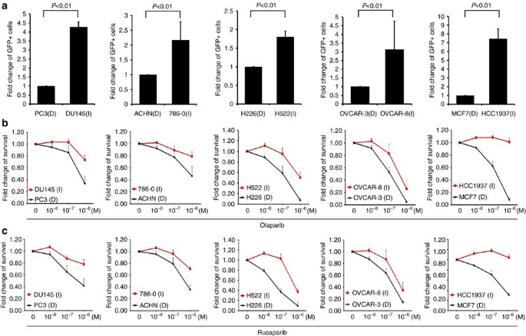Figure 2: The HRD gene signature predicts sensitivity to PARP inhibitors in cancer cells. (a) Modified HR repair assay was performed by transfecting cells with DR-GFP DSB substrate plasmid and I-SceI plasmid through electroporation at 270 V, 975uF using a Bio-Rad genepulsar II. Flow cytometry analysis was performed 48–72 h later to detect GFP-positive cells. Each value is shown as mean+s.d. for three independent experiments. Student’st-test showed increased HR repair efficiency in HR-intact cell lines compared with the HR-deficient cell lines in each cancer type, respectively. (b,c) Colony formation assay was performed with indicated concentrations of olaparib (b) or rucaparib (c). Each value is relative to the value in the cells treated with vehicle control. Results are shown as mean+s.d. from three independent experiments. Student’st-test showed that the drug response to PARP inhibitors differed between cancer cell lines with and without the HRD gene signature (P<0.05 throughb,c). Figure 2: The HRD gene signature predicts sensitivity to PARP inhibitors in cancer cells. ( a ) Modified HR repair assay was performed by transfecting cells with DR-GFP DSB substrate plasmid and I-SceI plasmid through electroporation at 270 V, 975uF using a Bio-Rad genepulsar II. Flow cytometry analysis was performed 48–72 h later to detect GFP-positive cells. Each value is shown as mean+s.d. for three independent experiments. Student’s t -test showed increased HR repair efficiency in HR-intact cell lines compared with the HR-deficient cell lines in each cancer type, respectively. ( b , c ) Colony formation assay was performed with indicated concentrations of olaparib ( b ) or rucaparib ( c ). Each value is relative to the value in the cells treated with vehicle control. Results are shown as mean+s.d. from three independent experiments. Student’s t -test showed that the drug response to PARP inhibitors differed between cancer cell lines with and without the HRD gene signature ( P <0.05 through b , c ). Full size image Having determined the association between the HRD gene signature and HR repair capacity in cancer cell lines, we then asked whether the changes of the HRD gene signature at the transcriptional levels are correlated with their changes at the protein level in cancer cells. To answer this question, we obtained the systematic proteomic profiling data through a mass spectrometry analysis from breast cancer cell lines, which are identified as HR-deficient or HR-intact cell lines by gene signature analysis. We then compared the difference of protein expression levels between HR-deficient and HR-intact cell lines ( Supplementary Table 2 ). The change at the protein level is closely correlated with the changes at the transcriptional level. In Supplementary Fig. 8 , we further showed that similar functional pathways and networks were identified from proteomic data analysis compared with the microarray data analysis ( Supplementary Fig. 2 ). Together, these data suggest that gene expression profile analysis may permit functional identification of HR deficiency without the need for identification of the specific genetic or epigenetic aberrations in the HR repair network and, more importantly, that the HRD gene signature may be used to predict the sensitivity of tumour cells to targeted therapeutics for HR deficiency such as PARP inhibitors. Reversal of HR deficiency in BRCA1 -depleted cells Surprisingly, our analyses showed that breast cancer cell line HCC1937, which has BRCA1 mutation, did not exhibit gene expression patterns similar to the HRD gene signature, did not exhibit HR repair deficiency, and did not exhibit increased sensitivity to PARP inhibitors compared with MCF-7 cells with wild-type BRCA1 ( Fig. 2a–c ). We suspect that due to impaired DNA repair, additional genetic alterations may accumulate in these BRCA1 -mutated cells that, in turn, restore HR repair deficiency. A recent study has reported that PTEN is frequently mutated in BRCA1 -deficient tumours, which is indeed mutated in HCC1937 (ref. 20 ). In light of these observations, we ask whether PTEN loss might affect HR repair in BRCA1 -deficient cells. We generated BRCA1 knockdown, PTEN knockdown and BRCA1-PTEN double-knockdown cells in the MCF-10A background and subjected these cell lines to microarray analysis. Expression of these genes was significantly reduced in the knockdown cells, and deficiency of these genes did not affect the cell cycle distribution under normal culture conditions ( Supplementary Fig. 9 ). Interestingly, cells with BRCA1 deficiency or PTEN deficiency formed a cluster with the HRD gene signature. However, BRCA1-PTEN double-knockdown cells, like HCC1937, had a gene signature similar to that of control cells ( Fig. 3a ), suggesting that co-concurrent loss of PTEN and BRCA1 could potentially restore the HR repair efficiency in cells with defection of either BRCA1 or PTEN gene alone. 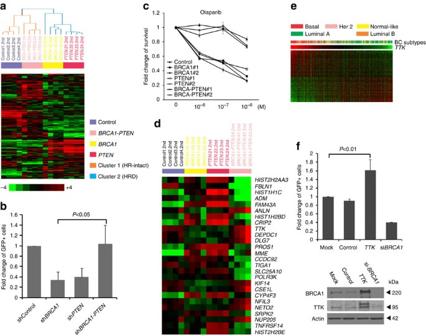Figure 3: Loss ofPTENreverses HRD and confers PARP inhibitor resistance toBRCA1-depleted cells through overexpression ofTTK. (a) MCF-10A cells were infected by the indicated lentiviral particles targeting the indicated genes. Control cells and knockdown cells were subjected to microarray analysis. The presence of the HRD gene signature was analysed by supervised clustering analysis. (b) Modified HR repair assay was performed in MCF-10A cells by transfecting cells with DR-GFP DSB substrate plasmid and I-SceI plasmid through electroporation, followed by analysis of GFP-positive cells by flow cytometry 48–72 h later. Student’st-test was performed from results of three independent experiments as mean+s.d. (c) The rate of cell survival in response to olaparib was determined by colony formation assay. Each value was relative to control cells without treatment and represents the mean±s.d. from three independent experiments. Student’st-test showed that treatment response differed betweenBRCA1-PTENdouble-knockdown cells and single-knockdown cells (P<0.001). (d) Heat map of the HRD gene signature with the 26 genes most significantly changed inBRCA1-PTENdouble-knockdown cells compared with single-knockdown cells. (e) Microarray data from 295 breast cancers were clustered into basal-like, Her2-positive (Her2), luminal A, luminal B and normal breast-like. Gene expression levels ofTTKamong the different breast cancer subtypes are indicated. (f) Quantitative analysis of HR repair assay in cells transfected withTTKplasmids. Results are shown as mean+s.d. from three independent experiments. Student’st-test showed that overexpression of TTK significantly increased HR repair efficiency (P<0.05).BRCA1SMARTpool siRNA was used as a positive control. Western blots demonstrating effective knockdown are shown to the bottom. Figure 3: Loss of PTEN reverses HRD and confers PARP inhibitor resistance to BRCA1 -depleted cells through overexpression of TTK . ( a ) MCF-10A cells were infected by the indicated lentiviral particles targeting the indicated genes. Control cells and knockdown cells were subjected to microarray analysis. The presence of the HRD gene signature was analysed by supervised clustering analysis. ( b ) Modified HR repair assay was performed in MCF-10A cells by transfecting cells with DR-GFP DSB substrate plasmid and I-SceI plasmid through electroporation, followed by analysis of GFP-positive cells by flow cytometry 48–72 h later. Student’s t -test was performed from results of three independent experiments as mean+s.d. ( c ) The rate of cell survival in response to olaparib was determined by colony formation assay. Each value was relative to control cells without treatment and represents the mean±s.d. from three independent experiments. Student’s t -test showed that treatment response differed between BRCA1-PTEN double-knockdown cells and single-knockdown cells ( P <0.001). ( d ) Heat map of the HRD gene signature with the 26 genes most significantly changed in BRCA1-PTEN double-knockdown cells compared with single-knockdown cells. ( e ) Microarray data from 295 breast cancers were clustered into basal-like, Her2-positive (Her2), luminal A, luminal B and normal breast-like. Gene expression levels of TTK among the different breast cancer subtypes are indicated. ( f ) Quantitative analysis of HR repair assay in cells transfected with TTK plasmids. Results are shown as mean+s.d. from three independent experiments. Student’s t -test showed that overexpression of TTK significantly increased HR repair efficiency ( P <0.05). BRCA1 SMARTpool siRNA was used as a positive control. Western blots demonstrating effective knockdown are shown to the bottom. Full size image To further test this possibility, we performed HR repair assays in the knockdown cell lines. As expected, BRCA1-PTEN double-knockdown cells showed an increase in HR repair efficiency (or restored HR repair efficiency) compared with BRCA1 or PTEN single-gene-knockdown cells ( Fig. 3b ). We then tested the sensitivity of these cells to PARP inhibitor. BRCA1 and PTEN deficiency alone sensitized cells to olaparib ( Fig. 3c ), consistent with previously reported functions of BRCA1 and PTEN in regulating HR repair [16] , [17] , [21] , [22] . However, as expected, BRCA1-PTEN double knockdown did not sensitize cells to PARP inhibitor treatment and indeed were indistinguishable from control cells. Collectively, these data strongly support the concept that additional genetic alterations such as loss of PTEN can reverse HR deficiency in BRCA1 -deficient cells, suggesting that analysis of genetic alterations in individual genes involved in HR repair may not reflect the overall functional status of the HR repair network. In contrast, the HRD signature can provide a functional assessment of HR repair status that integrates inputs from multiple upstream mediators. Next, we sought to investigate the molecular mechanism underlying the enhanced HR repair in BRCA1-PTEN double-knockdown cells. We identified 26 genes in the HRD gene signature that had the greatest differences in expression between BRCA1–PTEN double-knockdown cells and single-gene-knockdown cells, using a scoring system described in Methods ( Fig. 3d ). Among these candidate genes, we focused on kinases as they represent the most druggable targets for chemical modulation of the HR repair network. We found that expression level of the TTK protein kinase, that we initially cloned [23] , was downregulated in PTEN or BRCA1 single-gene-knockdown cells. However, TTK expression level was increased in BRCA1-PTEN double-knockdown cells ( Fig. 3d ). As co-mutations of BRCA1 and PTEN are frequently observed in basal-like breast cancer [20] , we analysed TTK expression in this breast cancer subtype. We found that TTK expression was significantly enriched in basal-like breast cancer compared with other breast cancer subtypes ( Fig. 3e ). In addition, we found that the basal-like breast cancer cell line, HCC1937, which contains both BRCA1 and PTEN mutations, had a higher TTK expression level than other breast cancer cell lines ( Supplementary Fig. 10a ). TTK is a dual-specificity protein kinase that can phosphorylate tyrosine, serine and threonine [23] . It is associated with cell proliferation and regulates chromosome alignment and segregation during mitosis [23] , [24] . However, it remains unknown whether TTK plays a direct role in DNA repair. Thus, we tested whether TTK regulates HR repair. As we expected, overexpression of TTK increased HR repair ( Fig. 3f ). These results suggested that increased expression of TTK may contribute to increased HR repair efficiency in BRCA1-PTEN double-knockdown cells. Moreover, TTK inhibitor AZ3146 enhanced olaparib-induced apoptosis in HCC1937 cells ( Supplementary Fig. 10b ). Altogether, these data demonstrated that concurrent loss of PTEN and BRCA1 might rewire the HR repair network through regulating the expression of key genes such as TTK , which may be responsible for PARP inhibitor resistance observed in clinical trials in basal-like breast cancer or TNBC carrying a high frequency of dysfunctional BRCA1 and PTEN [20] . Identification of PARP inhibitor-synergizing agents Given that the HRD gene signature can functionally link transcriptional changes to HR repair deficiency, we asked whether we could identify agents that would induce the HRD gene signature and thereby induce sensitivity of cancer cells to DNA damage-inducing treatment such as PARP inhibitors. To this end, we compared data from the Connectivity Map with the HRD gene signature. The Connectivity Map is a public database with a large number of drug-associated gene expression profiles [25] . We searched the database for agents that caused gene expression changes overlapping with the HRD gene signature and therefore might be expected to induce sensitivity to PARP inhibitors. Remarkably, we found that PI3K inhibitor LY-294002, mTOR inhibitor rapamycin, HDAC inhibitor vorinostat and Hsp90 inhibitor AUY922 were ranked near the top of the Connectivity Map list in terms of inducing the HRD gene signature-like gene expression profiles. We first used HR repair assay described above to directly determine the effects of LY-294002 and rapamycin on HR repair. Previous studies have shown that PI3K inhibitor and rapamycin treatment disrupt cell growth signalling and thereby lead to cell cycle arrest at G1 phase [26] . To exclude any indirect effect of cell cycle distribution on HR repair, we used contact inhibition ( Supplementary Fig. 11a ) and aphidicolin ( Supplementary Fig. 11b ), a DNA polymerase inhibitor, to block replication and assure same cell cycle distribution in the control cells and the cells treated with LY-294002 or rapamycin. As expected, LY-294002 and rapamycin significantly reduced HR repair efficiency in both conditions ( Fig. 4a,b ). These data supported the notion that LY-294002 and rapamycin indeed inhibit HR repair. To further assess whether these drugs could sensitize cancer cells to PARP inhibitors, we selected cancer cell lines of a variety of different cancer types that did not exhibit the HRD gene signature. The degree of synergy of drug combination in a fixed molar ratio was calculated with the combination index algorithm as previously described [27] . In general, CI<1 indicates synergy and CI>1 indicates antagonism. In the cell lines we tested, the combination of LY-294002 or rapamycin synergized with PARP inhibitor olaparib ( Fig. 4c , Supplementary Fig. 11c ) or rucaparib ( Fig. 4d , Supplementary Fig. 11d ). In addition, rapamycin combined with PARP inhibitors showed an even larger synergistic enhancement of growth inhibition as compared with LY-294002 with PARP inhibitors in the majority of cell lines tested. Consistent with these findings, recent reports have used different approaches to discover that PI3K inhibitors in combination with PARP inhibitor reduced tumour burden in a BRCA1 -deficient mouse model and sensitized BRCA -proficient tumours by impairing BRCA1/2 expression [28] , [29] . Furthermore, we have validated the synergistic effect of HDAC inhibitor vorinostat ( Supplementary Fig. 11e ) or Hsp90 inhibitor AUY922 ( Supplementary Fig. 11f ) on PARP inhibitor treatment in HCC1937 cells. We found a relatively higher synergy from AUY922 combinations as compared with vorinostat combinations. Hence, using the HRD gene signature as a drug discovery framework, we not only correctly predicted the previously reported therapeutic effect from the combination of a PI3K inhibitor [28] , [29] or Hsp90 inhibitor [30] with a PARP inhibitor, but also discovered that an mTOR inhibitor, or an HDAC inhibitor rendered cells sensitive to PARP inhibitor treatment and could be used to develop effective combination therapies that would benefit patients. In addition, the use of the HRD gene signature to efficiently identify drugs that inhibit HR repair provided additional strong evidence that the HRD gene signature is indeed functionally linked with HR deficiency. 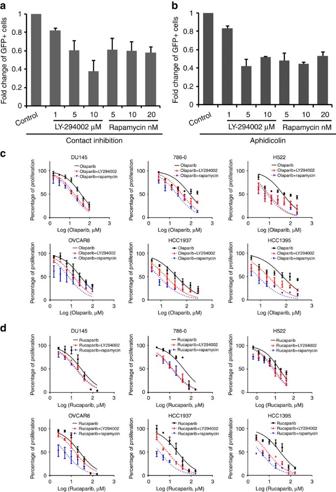Figure 4: Validation of agents synergizing with PARP inhibitors treatment predicted by the HRD gene signature. (a) U2OS cells were seeded at a high density to allow contact inhibition and transfected with I-SceI plasmid to induce DSBs. Then cells were treated with the indicated concentrations of PI3K inhibitor LY-294002 or mTOR inhibitor rapamycin for 16 h before analysis of GFP-positive cells. (b) U2OS cells were treated with the indicated concentrations of LY-294002 or rapamycin after I-SceI transfection and then treated with replication inhibitor aphidicoline (10 μM) to synchronize cell cycle for 16 h before the HR repair efficiency analysis. For bothaandb, results are shown as mean+s.d. from three independent experiments. Student’st-test (P<0.05). (c,d) The indicated cancer cell lines were treated with single or combined treatment of PARP inhibitor olaparib (c) or rucaparib (d), with LY-294002 or rapamycin and analysed by MTT assay. Each value is relative to the value in the cells treated with vehicle control. Results are shown as mean±s.e.m. from three independent experiments. The CI values calculated by CompuSyn software are listed inSupplementary Fig. 11c,d. Figure 4: Validation of agents synergizing with PARP inhibitors treatment predicted by the HRD gene signature. ( a ) U2OS cells were seeded at a high density to allow contact inhibition and transfected with I- Sce I plasmid to induce DSBs. Then cells were treated with the indicated concentrations of PI3K inhibitor LY-294002 or mTOR inhibitor rapamycin for 16 h before analysis of GFP-positive cells. ( b ) U2OS cells were treated with the indicated concentrations of LY-294002 or rapamycin after I- Sce I transfection and then treated with replication inhibitor aphidicoline (10 μM) to synchronize cell cycle for 16 h before the HR repair efficiency analysis. For both a and b , results are shown as mean+s.d. from three independent experiments. Student’s t -test ( P <0.05). ( c , d ) The indicated cancer cell lines were treated with single or combined treatment of PARP inhibitor olaparib ( c ) or rucaparib ( d ), with LY-294002 or rapamycin and analysed by MTT assay. Each value is relative to the value in the cells treated with vehicle control. Results are shown as mean±s.e.m. from three independent experiments. The CI values calculated by CompuSyn software are listed in Supplementary Fig. 11c,d . Full size image Prediction of clinical outcome in multiple human cancers In the next step, we used patient tumour samples to test whether the HRD gene signature correlates with clinical outcomes. We analysed four independent cancer data sets including breast, ovarian and lung cancers. We clustered patients hierarchically into two groups on the basis of similarity of gene expression profiles to the HRD gene signature. Among patients with breast and lung cancers, those with the HRD gene signature had better overall survival than those without the signature ( Fig. 5 ). In addition, we generated microarray data from 87 ovarian cancer patients, and these data showed results consistent with those in the breast and lung cancer data sets ( Supplementary Fig. 12 ). As we mentioned earlier, HR deficiency sensitizes cancer cells to DNA damaging inducing therapy, and thus the above observations may indicate the ability of the HRD gene signature to predict clinical outcomes as a result of different DNA damage-related treatments. 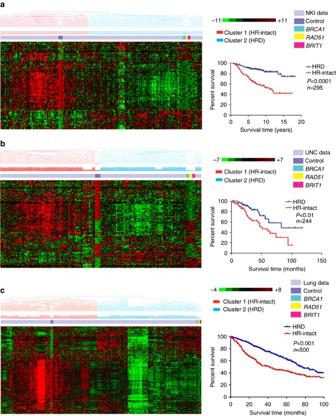Figure 5: The HRD gene signature predicts overall survival in independent breast and lung cancer patient cohorts. Data sets from patients with breast (a,b) and lung cancer (c) were clustered into two groups on the basis of whether the gene expression pattern was similar to the HRD gene signature. Kaplan–Meier overall survival curves are shown.P-values are from Log-rank test. Figure 5: The HRD gene signature predicts overall survival in independent breast and lung cancer patient cohorts. Data sets from patients with breast ( a , b ) and lung cancer ( c ) were clustered into two groups on the basis of whether the gene expression pattern was similar to the HRD gene signature. Kaplan–Meier overall survival curves are shown. P -values are from Log-rank test. Full size image Cells have evolved a complex DNA damage repair system, HR repair, which plays a fundamental role in maintaining genomic integrity and preventing tumorigenesis. Given the immense complexity of HR repair, identifying dysfunctional HR repair in human cancers is an enormous challenge. Instead of examining individual genes involved in HR repair, in this study, we used gene expression profiling to provide a global network view of the consequences of HR deficiency. Our data suggest that HR repair components are not independent. Instead, they form a network that is responsible for the integrated HR repair capacity of cells. Consistent with our findings from transcriptomic data, a recent quantitative proteomics profiling of poly (ADP-ribose) (pADPr)-associated protein complexes revealed complexity of the DNA damage response network in the context of poly(ADP-ribosyl)ation [31] , [32] . Interestingly, many genes in the HRD gene signature are potential pADPr-binding proteins identified from this study [32] . It is possible that many of these pADPr-binding proteins may exert a fine-tuned control of HR repair process, which may provide an additional rationale to use PARP inhibitors as adjunct to chemo/radiotherapy. Given the complexity of the HR repair network, the HRD gene signature allows interrogation of the status of HR repair by simultaneously considering hundreds of genes and thereby allows identification of HR deficiency in a given cellular state independent of underlying mechanism. The HR repair network is not static but rather dynamic during tumour evolution, which can be extensively rewired during tumour progression. As shown in our current study and previous reports, BRCA1/2 -mutated tumours may not necessarily be HR deficient because mutations in other genes can reverse HR deficiency through loss of PTEN or 53BP1 or by reversion of BRCA1/2 mutations [33] , [34] , [35] , [36] . As shown in our study, the combined effects of co-mutations/co-genetic alterations in cancer cells could be more determinative than the effects of individual alterations in terms of the functional behaviour of cancer cells. The phenotypes may not be the simple sum of each genetic change in cancer cells. With the advent of next-generation sequencing, we may be able to catalogue all the individual genetic alterations in a given tumour sample. However, to decipher the overall impact of these genetic alterations will likely require analyses of functional networks, which are perturbed by these genetic alterations from a systems biology level, instead of dissection of the functions of individual genetic alterations independently. In addition to biological insights, our data suggest that the HRD gene signature can be used as a potential prognostic tool for cancer patient outcome. Furthermore, we explored the potential therapeutic implications of the HRD gene signature. One of the recent most exciting therapeutic breakthroughs in cancer is the identification of a synthetic lethal interaction between HR deficiency and PARP inhibitors [16] , [17] . As a targeted therapeutic, the implementation of PARP inhibitors into patient management thus largely depends on accurate identification of patients with HR-deficient tumours as well as on approaches to prevent the emergence of resistance. The advantage of this HRD gene signature as a molecular assessment of HR deficiency without interrogating individual genetic alterations in cancer may allow us to develop practical and effective companion diagnostics able to robustly identify patients likely to benefit from PARP inhibitors beyond those with BRCA1/2 defects. Recent clinical trials of PARP inhibitors have shown poor response rate [37] , [38] , [39] in BRCA1/2 -deficient cancer patients, suggesting that only a portion of patients with BRCA1/2 mutants respond and unfortunately responses are usually short-lived. In our study, analysis of the HR repair network by gene expression profiling allowed us to identify chemicals targeting HR repair process. Our findings, together with the aforementioned recent reports confirming the therapeutic benefit of combining a PARP inhibitor with a PI3K inhibitor or an Hsp90 inhibitor [30] , suggest that combining TTK, mTOR, PI3K, HDAC or Hsp90 inhibitors with PARP inhibitors could also be promising approaches to improve responses to PARP inhibitor treatment, or more generally to DNA damage-inducing treatment such as radiation therapy and chemotherapy with cisplatin. It is worthy of noting that a recent study showed that PARP-1 inhibition leads to activation of mTORC1 complex due to reduced AMPK activity [40] . This result together with our findings strongly suggest that the therapeutic benefit of combining PARP inhibitor with mTOR inhibitor may be mediated by targeting both HR repair pathway and the PARP inhibitor-induced suppression of AMPK pathway. Cell culture and reagents U2OS cells (American type culture collection, ATCC) were maintained in McCoy’s 5A medium supplemented with 10% fetal bovine serum. MCF-10A cells (ATCC) were cultured in mammary epithelial growth medium containing insulin, hydrocortisone, epidermal growth factor and bovine pituitary extract (Clonetics). EVSAT cells (Creative Bioarray, NY, USA) were cultured in MEM containing 10% fetal bovine serum. MDA-MB-436 cells (ATCC) were maintained in DMEM medium supplemented with 10% fetal bovine serum. PC3, DU145, ACHN, 786-0, H226, H522, OVCAR-3, OVCAR-8 and MCF-7 cells were all obtained from ATCC and maintained according to ATCC instructions. BRCA1 (D-9) monoclonal and TTK polyclonal antibodies were purchased from Santa Cruz (SC-6954, 1:1,000) and Cell Signaling (#3255, 1:1,000), respectively. ZNF668 antibodies were generated as previously described [41] . Uncropped scans of the most important western blots are listed as supplementary figures in Supplementary Fig. 13 . PI3K inhibitor LY-294002 and mTOR inhibitor rapamycin were purchased from Sigma. PARP inhibitors olaparib and rucaparib, HDAC inhibitor vorinostat and Hsp90 inhibitor AUY922 were from Selleckchem. TTK inhibitor AZ3146 was purchased from R&D Systems. Lentiviral infection and plasmid siRNA transfection MCF-10A cells were infected with individual MISSION lentiviral particles (Sigma) targeting BRCA1 , RAD51 , BRIT1 , PTEN , ATM , ATR , 53BP1 , CHK1 , CHK2 or BRCA2 according to the manufacturer’s instructions. After infection, cells with stable knockdown were selected by using puromycin (1 μg ml −1 ) for 10–15 days. For transient transfection, TTK or BRCA1 was knocked down using SMARTpool siRNAs (Dharmacon) and ZNF668 knocked down by the ON-TARGET-plus ZNF668 siRNA (Dharmacon). TTK cDNA was purchased from Harvard Plasmid Core and subcloned using Gateway technology (Invitrogen). In U2OS cells, siRNAs were transfected with oligofectamine (Invitrogen), and plasmid was transfected with FuGENE 6 (Roche). In MCF-10A cells, transfection of plasmids was performed with lipofectamine 2000 (Invitrogen). All small hairpin RNA/siRNA sequences are described in Supplementary Table 3 . Microarray analysis Microarray analysis was conducted as previously described [42] . Total RNA was extracted using a mirVana RNA isolation labelling kit (Ambion). We used 500 ng of total RNA for labelling and hybridization based on the manufacturer’s procedures (Illumina). Sentrix Human6 v2 Expression Bead Chip and HumanHT-12 v4 Expression Beadchip were used. The bead chips were scanned with a BeadArray Reader (Illumina). After normalization with the Linear Models for Microarray Data (LIMMA) package in the R language environment and log2 transformation, array data were subjected to further analysis. Primary microarray data are available in the National Center for Biotechnology Information Gene Expression Omnibus public database (Illumina platform, GEO accession number GSE54269 ). The random variance t- test was used to identify genes differentially expressed between the two classes that were compared using BRB-ArrayTools [43] . The random variance t- test is an improvement over the standard separate t -test as it allows information to be shared among genes about within-class variation without assuming that all genes have the same variance. Gene expression differences were considered significant if P <0.001. Gene set enrichment analysis was performed using Ingenuity Pathway Program (version 12710793). To define the genes that most significantly changed in BRCA1 (a), PTEN (b) and double-knockdown cells (c), a score was signed to each gene using the following formula after their expression levels were compared with expression levels in control cells as described in previous paper [44] : a/c+b/c≤1.2 for genes overexpressed in c; c/a+c/b≤1.2 for genes underexpressed in c. HR repair analysis A schematic diagram of HR repair assay is shown in Supplementary Fig. 1a . DR-GFP, pCAGGS and pCBASce plasmids were kindly provided by Dr Maria Jasin (Memorial Sloan-Kettering Cancer Center, New York, NY). U2OS cells containing a single copy of the HR repair reporter substrate DR-GFP in a random locus were generated as previously described [12] . GFP-expressing plasmid (pEGFP-C1) was used for transfection efficiency control. Twenty-four hours after ZNF668 siRNA, TTK plasmid or BRCA1 siRNA transfection, cells were re-seeded; the next day, cells were transfected with pCBASce plasmids. For cell lines that do not stably contain the DR-GFP plasmid, 1 × 10 6 cells were electroporated with 12 μg of DR-GFP and 12 μg of pCBASce plasmids at 270 V, 975uF using a Bio-Rad genepulsar II [45] . About 48–72 h later, flow cytometry analysis was performed to detect GFP-positive cells using a FACScalibur apparatus with CellQuest software (Becton Dickinson, San Jose, CA). Unless otherwise specified, results were mean+s.d. from three independent experiments. Flow cytometry analysis Cells were fixed with 70% cold ethanol (−20 °C) overnight and then resuspended in staining solution (10 μg ml −1 propidium iodide, 20 μg ml −1 RNAase A and 0.05% Triton X-100). Cell cycle analysis was performed at the MD Anderson Cancer Center Flow Cytometry and Cellular Imaging Facility. Any given analyses were repeated at least three times. Colony formation assay Cells were seeded at low density and treated with indicated concentrations of drugs the next day; cells were then left for 2 weeks to allow colonies to form. Colonies were stained with staining solution (0.25% crystal violet, 25% methanol in 1 × phosphate-buffered saline) for colony visualization. Colonies were counted manually (colonies containing 50 or more cells were counted) or digitally using ImageJ software with customized parameters optimized based on three preliminary manual counts or blindly chosen. Unless otherwise stated, each value is relative to the value in the cells treated with vehicle control. Results are shown as mean+s.d. from three independent experiments. Cell proliferation assay Cell proliferation was measured by MTT (Sigma) reduction. To test the cell proliferation rate, cells were seeded in 96‐well plates in a total volume of 100 μl in triplicate in each experiment. The next day, cells were treated with indicated concentrations of drugs. Five days later, 20 μl of MTT substrate (2 mg ml −1 ) was added to each well and incubated with cells for 3 h. Then the culture medium was removed, and 100 μl of dimethyl sulphoxide was added. Plates were read at 490 and 650 nm (background) in a microplate reader (Molecular Devices). After subtraction of background, the cell viability was calculated as fold change relative to control cells. The OD values were analysed with Graphpad Prism 6.0 software. Each value is relative to the value in the cells treated with vehicle control. Results are shown as mean±s.e.m. from three independent experiments. Drug combination studies Drug combination treatments results were obtained from MTT assays of at least three replications and the combination index was calculated by CompuSyn software using the Chou-Talalay equation, which takes into account both the potency (IC50) and the shape of the dose-effect curve [46] . CI<1 indicated synergism, and CI=1 and CI>1 indicated additive and antagonism, respectively. Survival analysis Two independent data sets of breast cancer patients, the Netherlands Cancer Institute (NKI) [47] and University of North Carolina (UNC) [48] cohorts, one data set of lung cancer patients and one data set of ovarian cancer patients containing both genome-wide expression data and patient survival data were used for survival analysis. Kaplan–Meier analysis and the Log‐rank test were used to estimate patient prognosis. Statistical analysis All statistical analysis was performed with a one-tailed Student’s t -test. Accession codes: The microarray data have been deposited in the Gene Expression Omnibus Database under accession code GSE54269 . How to cite this article : Peng, G. et al. Genome-wide transcriptome profiling of homologous recombination DNA repair. Nat. Commun. 5:3361 doi: 10.1038/ncomms4361 (2014).